Forecasting flowering phenology under climate warming by modelling the regulatory dynamics of flowering-time genes Understanding how climate warming has an impact on the life cycle schedule of terrestrial organisms is critical to evaluate ecosystem vulnerability to environmental change. Despite recent advances identifying the molecular basis of temperature responses, few studies have incorporated this knowledge into predictive models. Here we develop a method to forecast flowering phenology by modelling regulatory dynamics of key flowering-time genes in perennial life cycles. The model, parameterized by controlled laboratory experiments, accurately reproduces the seasonal changes in gene expression, the corresponding timing of floral initiation and return to vegetative growth after a period of flowering in complex natural environments. A striking scenario forecast by the model under climate warming is that the shift in the return time to vegetative growth is greater than that in floral initiation, which results in a significant reduction of the flowering period. Our study demonstrates the usefulness of gene expression assessment to predict unexplored risks of climate change. Life cycle schedules of diverse species are often triggered by temperature-related cues, and significant changes in biological systems occur under the influence of warming temperatures [1] . Ecological studies have suggested the phenological shifts in the key life history events of wild plants and animals in response to climate warming [2] , [3] , [4] , [5] . Recently, the molecular genetics underpinning temperature responses has been uncovered in laboratory-based model systems [6] , [7] , [8] . Considering the threat to global biodiversity, the application of ample molecular genetic data in the laboratory to real environmental problems outside the laboratory offers advantages for the genetically informed assessment of ecosystem vulnerability to climate change [9] , [10] . Despite its critical importance, our understanding of the molecular mechanism underlying the rapid phenological changes observed in nature is limited. Here we develop a predictive model that incorporates gene-regulatory dynamics involved in a representative phenological event, namely flowering time, to forecast plant phenology in complex natural environments. In a previous study, we showed that FLOWERING LOCUS C ( FLC ), a MADS-domain-containing transcription factor [11] , [12] , has an important role in monitoring the seasonal temperature trends in a fluctuating natural environment in Arabidopsis halleri subsp. gemmifera, a perennial relative of the annual A. thaliana [13] . A. halleri is characterized by the formation of aerial rosettes on apical and lateral meristems following flowering ( Fig. 1a ). This perennial life cycle adds interesting complexity to the study of flowering phenology—the timing of the return to vegetative growth. In annual plants, flowering is irreversible, leading to fruiting and plant death. However, perennials are characterized by a reversion to vegetative growth (hereafter, ‘reversion’) after a period of flower development. We study this reversible reproductive feature of perennials by focusing on the key temperature-dependent pathway to flowering—the transcriptional regulation of two vernalization-specific genes ( VERNALIZATION-INSENSITIVE 3 : AhgVIN3 and AhgFLC ) [11] , [12] , [13] , [14] , [15] and one floral integrator gene ( FLOWERING LOCUS T : AhgFT ) [16] , [17] in A. halleri . We selected two natural populations of A. halleri : Hyogo and Hakodate ( Fig. 1b ). The Hyogo population has been previously studied [13] , and the Hakodate population was newly added to examine the applicability of the model to independent populations. 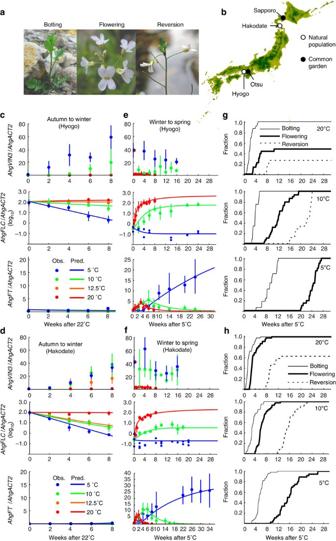Figure 1: Gene expression analysis in the laboratory-based system usingA. halleri. (a) Bolting, flowering and reversion ofA. halleri.(b) Locations of the natural habitats of the Hyogo and Hakodate populations and two common gardens (Otsu and Sapporo) for the reciprocal transplant experiments. Observed (mean±s.d. of three replicates) and predicted (lines) expression levels ofAhgVIN3, AhgFLCandAhgFTduring the temperature change from autumn to winter in the Hyogo population (c) and in the Hakodate population (d), and from winter to spring in the Hyogo population (e) and in the Hakodate population (f). At 5 °C, the raw data were plotted as small dots after removing unmeasurable data points. (g) Phenology of the Hyogo population. All plants bolted at 20 °C, but only 50% flowered and 25% reverted to vegetative growth because flower stems did not develop properly. (h) Phenology of the Hakodate population. Figure 1: Gene expression analysis in the laboratory-based system using A. halleri . ( a ) Bolting, flowering and reversion of A. halleri. ( b ) Locations of the natural habitats of the Hyogo and Hakodate populations and two common gardens (Otsu and Sapporo) for the reciprocal transplant experiments. Observed (mean±s.d. of three replicates) and predicted (lines) expression levels of AhgVIN3, AhgFLC and AhgFT during the temperature change from autumn to winter in the Hyogo population ( c ) and in the Hakodate population ( d ), and from winter to spring in the Hyogo population ( e ) and in the Hakodate population ( f ). At 5 °C, the raw data were plotted as small dots after removing unmeasurable data points. ( g ) Phenology of the Hyogo population. All plants bolted at 20 °C, but only 50% flowered and 25% reverted to vegetative growth because flower stems did not develop properly. ( h ) Phenology of the Hakodate population. Full size image The model is parameterized by the long-term gene expression dynamics monitored under controlled laboratory conditions. When the model is applied to transplant experiments in the field, it successfully reproduced the seasonal changes in gene expression and predicted the corresponding timing of floral initiation and reversion to vegetative growth in complex natural environments with exceptional accuracy. The model predicts that an increase in temperature of 4.5–5.3 °C would completely prevent this perennial plant from flowering. Given the conservation in the genetic network that regulates flowering across plant species, our approach can be applied to other plant species and would be of benefit in assessing the unexplored risks of climate change. Temperature manipulation experiments in the laboratory To obtain the long-term gene expression data essential for model construction and parameter fitting, we first used plants from the two populations in laboratory experiments. In the laboratory, we imitated two seasonal transitions in temperature—autumn to winter (AW) and winter to spring (WS)—under long-day conditions (16 h light/8 h dark). In the AW experiment, the plants were exposed to temperature changes from warm (22 °C) to three different levels of cold (5, 10 and 12.5 °C) and control (20 °C) conditions. The AhgVIN3 , AhgFLC and AhgFT mRNA levels were measured for 8 weeks after the exposure to 22 °C. In the Hyogo population, the expression of AhgVIN3 was not induced at 12.5 and 20 °C but increased gradually at a greater rate at lower temperatures ( Fig. 1c ), consistent with previous observations in annual Arabidopsis [18] . The AhgFLC mRNA levels declined gradually, at a greater rate at lower temperatures, although they were high at 12.5 and 20 °C ( Fig. 1c ). The Hakodate plants behaved similarly, except that AhgVIN3 was induced and AhgFLC was suppressed even at 12.5 °C ( Fig. 1d ). The AhgFT mRNA levels were low in both populations irrespective of the temperature condition ( Fig. 1c,d ). In the WS experiment, the plants were exposed to temperature changes from prolonged cold (10 weeks at 5 °C) to two warmer conditions (10 and 20 °C) and one control (5 °C) condition, and the mRNA levels of the same genes were monitored for 34 weeks after the prolonged cold exposure. In the Hyogo population, the AhgVIN3 mRNA levels decreased rapidly at 10 and 20 °C ( Fig. 1e ), consistent with the behaviour in A. thaliana [15] . The AhgFLC expression recovered gradually with a greater rate at warmer temperatures (10 and 20 °C; Fig. 1e ), which is characteristic of perennials of Brassicaceae [13] , [19] . The AhgFT expression was induced immediately after prolonged cold but was suppressed again earlier at warmer temperatures, resulting in a transient expression peak (10 and 20 °C; Fig. 1e ). At 5 °C, AhgVIN3 was continuously expressed at high levels, the AhgFLC mRNA levels remained low, and the AhgFT mRNA levels increased continuously ( Fig. 1e ). The Hakodate plants revealed a similar temperature dependence, except for the significantly high expression of AhgVIN3 even at 10 °C ( Fig. 1f ). There were clear delays in flowering phenology at lower temperatures. In the Hyogo population, bolting (a signal of floral initiation by elongation of flower stems; Fig. 1a ) and flowering occurred 48 and 135 days later at 5 °C than at 20 °C ( Fig. 1g , Supplementary Table S1 ), and this delay coincided with the delayed activation of AhgFT ( Fig. 1e ). The timing of reversion was also delayed at lower temperatures, and reversion did not occur at 5 °C ( Fig. 1g , Supplementary Table S1 ), suggesting the necessity of AhgFLC recovery and AhgFT suppression for reversion. As a result, the plants continued flowering for longer periods of time at a lower temperature. Overall, the Hakodate plants behaved similarly ( Fig. 1h ). A model integrating vernalization and photoperiod pathways The gene expression data obtained in the controlled laboratory conditions were then used to construct and parameterize a model that describes the regulatory relationship between AhgFLC and AhgFT under the influence of temperature and photoperiod ( Fig. 2a , Supplementary Tables S2–S5 ). The model was represented by ordinary differential equations, where the form of the equations reflected the known molecular interactions in Arabidopsis and gene-specific functions of temperature response ( Fig. 2b,c ) estimated using the data obtained in the above experiments. There were two important differences in the temperature response between AhgFLC and AhgFT . First, the production rates of two genes are both increasing functions of temperature, but the rate of increase is larger in AhgFLC than in AhgFT ( Fig. 2b,c ). The second difference was found in the temperature response of degradation rate. The degradation rate of AhgFLC decreased as the temperature rose ( Fig. 2b ), which allows the elevated accumulation of AhgFLC transcripts with the temperature increase. In contrast, the degradation rates of AhgFT increased with rising temperature ( Fig. 2c ), maintaining the stationary levels of the AhgFT transcript almost constant under most temperature ranges. These differences could have a critical role in regulating the flowering phenology under climate warming. 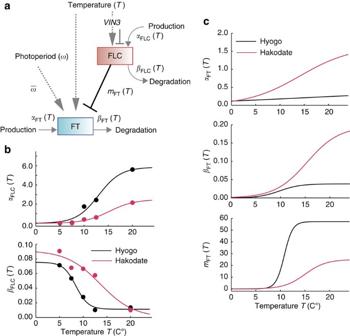Figure 2: Model illustration and gene-specific temperature response functions. (a) Scheme of the model.represents the critical photoperiod above which theAhgFTtranscript is produced. (b) Temperature response functions for production and degradation rates of theAhgFLCtranscript at the tissue level (αFLC(T) andβFLC(T)). (c) Temperature response functions for the production and degradation rates of theAhgFTtranscript at the tissue level (αFT(T) andβFT(T)) and the dissociation constants ofAhgFTrepression byAhgFLC(mFT(T)). Figure 2: Model illustration and gene-specific temperature response functions. ( a ) Scheme of the model. represents the critical photoperiod above which the AhgFT transcript is produced. ( b ) Temperature response functions for production and degradation rates of the AhgFLC transcript at the tissue level ( α FLC ( T ) and β FLC ( T )). ( c ) Temperature response functions for the production and degradation rates of the AhgFT transcript at the tissue level ( α FT ( T ) and β FT ( T )) and the dissociation constants of AhgFT repression by AhgFLC ( m FT ( T )). Full size image The model successfully explained the dynamics of AhgFLC and AhgFT expressions under various temperature conditions manipulated in the laboratory ( Fig. 1c–f ), which facilitates the prediction of the expression dynamics of these genes under arbitrary temperature conditions in nature. In addition to temperature, another important environmental signal that regulates FT is the photoperiod [9] . We incorporated a critical photoperiod parameter above which the AhgFT transcript is produced ( Fig. 2a ), and estimated the value by reciprocal transplant experiments (11.1 h for Hyogo and 11.3 h for Hakodate plants; Supplementary Fig. S1 ). We simulated the AhgFLC and AhgFT expressions based on the model and then forecasted the flowering phenology in a dynamically changing natural environment by attributing the simulated AhgFT expression levels to the timing of the phenological events. The expression levels of AhgFT on the onset dates of bolting and reversion were determined using the data obtained in the above laboratory experiments and the model ( Supplementary Table S6 ). Transplant experiments in complex natural environments To evaluate the usefulness of the model to forecast flowering phenology in nature, we performed reciprocal transplant experiments in two common gardens, Otsu (South site) and Sapporo (North site; Fig. 1b ), which are close to the Hyogo and Hakodate natural populations, respectively. At the South site, we monitored the AhgFLC and AhgFT mRNA levels for each population for one year from September 2011. When the model was applied to the plants under natural temperature and photoperiod conditions at the South site, the AhgFLC expression levels were predicted to decrease gradually from December in response to the temperature decline and start recovering in spring as the temperature increased in both populations ( Fig. 3a,b ). These predictions accurately accounted for the observations from the transplant experiments ( R 2 =0.87 for Hyogo and 0.90 for Hakodate plants). The dynamics of AhgFT were predicted using the estimated critical photoperiod parameter for each population after confirming that the difference in sampling time between the laboratory and common garden experiments does not influence the AhgFT expression measurements ( Supplementary Fig. S2 ). The model reproduced the observed dynamics of AhgFT expression, showing a transient peak in April, with exceptional accuracy ( Fig. 3a,b ; R 2 =0.76 for Hyogo and 0.92 for Hakodate plants). Moreover, the predicted timing of bolting and reversion were in good agreement with the observed phenology ( Fig. 3a,b ). The accurate prediction of flowering phenology in nature by the laboratory-based model contrasts sharply with previous studies [20] , [21] that have demonstrated the different behaviours of model species between laboratory and natural conditions. 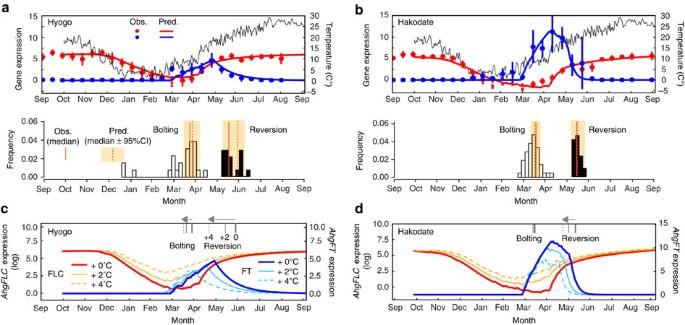Figure 3: Gene expression analysis in the South common garden and forecasted gene expression dynamics under warming. Observed (mean±s.d. of five replicates) and predicted (lines)AhgFLC(red; natural logarithmic scale) andAhgFT(blue) expression and the timing of bolting and reversion in the Hyogo population (a) and in the Hakodate population (b) transplanted at the South common garden (Otsu). The observed levels ofAhgFLCexpression were rescaled to have the same stationary state (calculated as the mean in September) under the laboratory conditions at 20 °C (Supplementary Table S2). The observed levels ofAhgFTexpression were rescaled to have the same maximum as the predicted value. Black lines represent the mean daily soil surface temperature. Orange vertical lines indicate the medians of observed (solid) and predicted (dashed) timings of bolting and reversion. Orange squares represent the predicted range (95% CI of median). Given the uncertainty in the relationship between theAhgFTexpression and phenotypic output, the 95% CI of median was calculated by bootstrapping based on 1,000 replications using the data inSupplementary Table S6. The predicted transcript levels under warming in the Hyogo population (c) and in the Hakodate population (d). 0 °C corresponds to the daily soil surface temperature monitored at the South common garden from October 2011 to September 2012. Grey vertical lines represent the predicted timing of bolting and reversion for three warming scenarios (0, 2, and 4 °C increase of temperature). Figure 3: Gene expression analysis in the South common garden and forecasted gene expression dynamics under warming. Observed (mean±s.d. of five replicates) and predicted (lines) AhgFLC (red; natural logarithmic scale) and AhgFT (blue) expression and the timing of bolting and reversion in the Hyogo population ( a ) and in the Hakodate population ( b ) transplanted at the South common garden (Otsu). The observed levels of AhgFLC expression were rescaled to have the same stationary state (calculated as the mean in September) under the laboratory conditions at 20 °C ( Supplementary Table S2 ). The observed levels of AhgFT expression were rescaled to have the same maximum as the predicted value. Black lines represent the mean daily soil surface temperature. Orange vertical lines indicate the medians of observed (solid) and predicted (dashed) timings of bolting and reversion. Orange squares represent the predicted range (95% CI of median). Given the uncertainty in the relationship between the AhgFT expression and phenotypic output, the 95% CI of median was calculated by bootstrapping based on 1,000 replications using the data in Supplementary Table S6 . The predicted transcript levels under warming in the Hyogo population ( c ) and in the Hakodate population ( d ). 0 °C corresponds to the daily soil surface temperature monitored at the South common garden from October 2011 to September 2012. Grey vertical lines represent the predicted timing of bolting and reversion for three warming scenarios (0, 2, and 4 °C increase of temperature). Full size image At the North site, we started monitoring in April 2012 because the ground was covered with dense snow during the winter. During the spring (26 April–31 May), the mean soil surface temperature at the North site was 2.69 °C lower than that at the South site. Because of the lower temperature, AhgFL C recovery and AhgFT suppression were predicted to occur later than at the South site, resulting in a delayed reversion time in both populations ( Fig. 4 ). These predictions were again in good agreement with the observations ( R 2 for AhgFLC and AhgFT , respectively, were 0.72 and 0.86 for Hyogo and 0.96 and 0.88 for Hakodate plants). The plants at the North site bolted 1 week after snowmelt ( Fig. 4 ), which was an ~5-week delay compared with the plants at the South site, but the direct effect of temperature on this delay was unclear because of the snow. 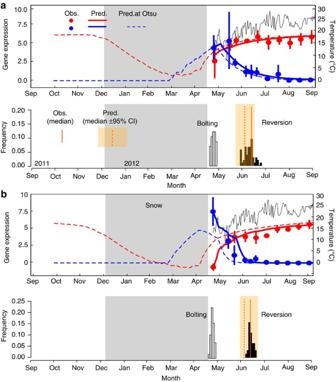Figure 4: Gene expression analysis in the North common garden. Observed (mean±s.d. of five replicates) and predicted (lines)AhgFLC(red; natural logarithmic scale) andAhgFT(blue) expression and the timing of bolting and reversion in the Hyogo population (a) and in the Hakodate population (b) transplanted at the North common garden (Sapporo). The predictions at the South common garden (Otsu) were also plotted as dashed lines. The same rescaling values were used for the South and North common gardens. Black lines represent the mean daily soil surface temperature. Orange vertical lines indicate the medians of observed (solid) and predicted (dashed) timings of bolting and reversion. Orange squares represent the predicted range (95% CI of median). The ground was covered with snow during the period shown by the shading. Figure 4: Gene expression analysis in the North common garden. Observed (mean±s.d. of five replicates) and predicted (lines) AhgFLC (red; natural logarithmic scale) and AhgFT (blue) expression and the timing of bolting and reversion in the Hyogo population ( a ) and in the Hakodate population ( b ) transplanted at the North common garden (Sapporo). The predictions at the South common garden (Otsu) were also plotted as dashed lines. The same rescaling values were used for the South and North common gardens. Black lines represent the mean daily soil surface temperature. Orange vertical lines indicate the medians of observed (solid) and predicted (dashed) timings of bolting and reversion. Orange squares represent the predicted range (95% CI of median). The ground was covered with snow during the period shown by the shading. Full size image Forecasting flowering phenology under climate changes To assess the impact of climate warming on the flowering phenology, we first simulated the seasonal changes in the AhgFLC and AhgFT expression when the temperature rises from the original level monitored at the South site from October 2011 to September 2012. Under warming conditions, the level of AhgFLC expression declined more slowly in winter, and recovery occurred earlier in spring in both populations ( Fig. 3c,d ). In response to the early recovery of AhgFLC , the timing of AhgFT suppression was significantly advanced, which resembled the observations in the laboratory (10 and 20 °C; Fig. 1e,f ). However, the timing of AhgFT activation was less affected by warming ( Fig. 3c,d ). As a result, warming by 2 °C (4 °C) advanced the timing of reversion by 16 (40) days, whereas it advanced the bolting timing by only 7 (11) days in the Hyogo population ( Fig. 3c ). In cases where the two genes responded similarly to the temperature change, the asymmetric response between bolting and reversion timing was less pronounced ( Supplementary Fig. S3 ). This result implies that the asymmetric phenological shift can be caused by the different temperature response between AhgFLC and AhgFT ( Fig. 2b,c ). Given the simulated dynamics of AhgFT expression, we forecasted the flowering phenology under a wide range of temperatures. As the temperature increased, both the bolting and reversion times advanced, but the shift in the reversion time was significantly greater ( Fig. 5a ). Because of this asymmetric response, the duration of flowering decreased gradually with warming ( Fig. 5b ). Additionally, the Hyogo plants were expected to lose the opportunity to flower when the temperature increased by 4.5 °C ( Fig. 5b ). The Hakodate plants were more robust, but they were also expected to be flowerless at 5.3 °C warming ( Fig. 5b ). This striking result implies the potentially high vulnerability of natural populations of A. halleri to climate warming, although the effect of increased temperature on survival and growth rates should be studied for a more comprehensive understanding. 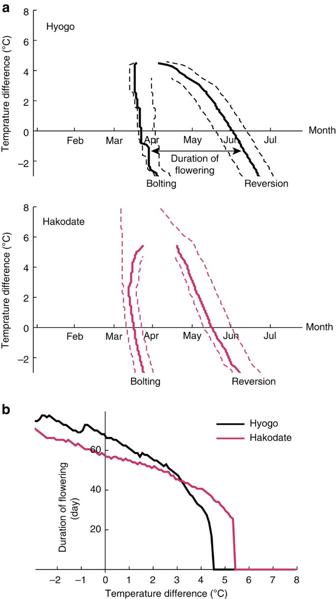Figure 5: Forecasted phenological shifts under a wide range of temperatures. Forecasted timing of bolting and reversion in the Hyogo and Hakodate populations (a) and flowering duration (b). Median (solid line) and the 95% CI of median (dashed line) are plotted. 0 °C corresponds to the daily soil surface temperature monitored at the South common garden (Otsu) from October 2011 to September 2012. Figure 5: Forecasted phenological shifts under a wide range of temperatures. Forecasted timing of bolting and reversion in the Hyogo and Hakodate populations ( a ) and flowering duration ( b ). Median (solid line) and the 95% CI of median (dashed line) are plotted. 0 °C corresponds to the daily soil surface temperature monitored at the South common garden (Otsu) from October 2011 to September 2012. Full size image Although the genetic mechanism of the flowering response to seasonal cues has been explored extensively, few studies have taken advantage of molecular approaches to understand the phenology shifts currently occurring in natural and agricultural systems. Our study shows that a seemingly complex trait, flowering phenology, can be modelled successfully based on the regulatory dynamics of a surprisingly small number of genes. Despite its simplicity, the model accurately predicted complex phenological responses to climate warming in a dynamically changing natural environment, which would offer advantages for systematic conservation planning. Our approach can be applied to crop species that have tightly interlinked vernalization and photoperiod pathways, such as wheat and barley, and will benefit the vulnerability assessment of an important ecosystem service, food production, on which human societies depend. Study species and laboratory experiments A. halleri (L.) O’Kane & Al-Shehbaz subsp. gemmifera (Matsum.) O’Kane & Al-Shehbaz is distributed in the Russian Far East and East Asia [22] . We collected 10 individuals from two natural populations. One was located in Hyogo in central Honshu (along the Omoide River, Taka-cho; 35°06' N, 134°55' E, alt. 190–230 m) and the other in Hakodate on Hokkaido, a northern island of Japan (along the Matsukura River, Hakodate City; 41°47' N, 140°49' E, alt. 10 m; see Fig. 1b ). The mean air temperatures were 16.8 °C in Hyogo and 9.1 °C in Hakodate (Japan Meteorological Agency 1981–2010). Because it was difficult to prepare genetically uniform seeds of this self-incompatible species, we grew the plants in continuous white fluorescent light at 22 °C until clonal reproduction (formation of aerial rosettes) and collected aerial rosettes of about 3 cm from the parent lines after flowering and reversion. The aerial rosettes were planted on the surface of a 7.5-cm-diameter pot containing a 6:1 (v/v) mixture of vermiculite and culture soil. The plants were then grown in continuous white fluorescent light at 22 °C for 6–8 weeks. Fully matured rosettes with average diameters of 7.31±0.11 cm were allocated to autumn–winter (AW) and winter–spring (WS) experiments. Three parent lines were chosen for the experiment. Individuals in the AW group were placed in an incubator (LH-80CCFL-6CT; NK Systems, Osaka, Japan) at four different temperatures (5, 10, 12.5, and 20 °C) under long-day conditions (18 h light/6 h dark) at a photon flux density of 50 μmol m −2 s −1 . The WS group was first placed at 5 °C for 10 weeks in an incubator (LP-130-E; NK Systems) under the same long-day photoperiod and then moved to an incubator (LH-80CCFL-6CT; NK Systems) at three different temperatures (5, 10, and 20 °C) under the same photoperiod conditions. We used 12–50 plants for each temperature condition and sampled young leaves of these plants once every 1 or 2 weeks, with three replicates at the same time (4 h after dawn). For long-term monitoring at 5 °C, the sampling interval was set as long as 4–12 weeks. Essentially, we changed the plants for each sampling to obtain a robust trend in gene expression, but several plants were sampled twice. The leaf samples were immediately preserved in liquid nitrogen and stored at −80 °C until RNA extraction. We recorded the dates of onset of bolting, flowering and reversion. The onset of bolting was defined as the elongation of flower stems past 2.0 cm. The onset of reversion was defined as the formation of aerial rosettes larger than 0.5 cm (diameter) on apical or lateral meristems. Aerial rosettes were not always produced, and basal rosettes developed new leaves after flowering. The same plants that were sampled for gene expression analysis were also used for phenology monitoring. To ensure a sufficiently large sample size, we also added new plants for phenology monitoring that had not been used for gene expression analysis. After the AW experiment, plants were returned to 22 °C under the same long-day conditions. Plants placed at 20 °C in the AW experiment remained in the vegetative stage for more than a year. Transplant experiments Fully mature rosette-oriented plants from five parent lines for each population were used for the transplant experiments at two common gardens. The South site (Otsu) was located in central Japan (the common garden in the Center of Ecological Research, Kyoto University, Otsu City, 34°58′ N, 135°57′ E, alt. 150 m), and the North site (Sapporo) was located in northern Japan (the common garden on the campus of Hokkaido University, Sapporo, 43°4′N, 141°20′E, alt. 15 m; Fig. 1b ). The plants were transferred to 18 cm diameter pots and directly buried on the ground surface (7 September and 2 August 2011, for the South and North sites, respectively). The pots were placed at least 20 cm apart to minimize competition among the plants. The soil consisted of a coarse-grained loamy soil in the lower half of the pot and a 1:1 mixture of fine-grained pumice and peat in the upper half. We also added a slow-acting fertilizer (MagAmp K) according to the manufacturer’s instructions (50 g per 12 l mixed soil). At the South site, the ambient temperature in the summer was high. Thus, plants first assimilated to high ambient temperatures in a growth chamber (CfER custom model; Nippon Medical & Chemical Instruments, Osaka, Japan) at 28 °C/25 °C under the long-day photoperiod (18 h light/6 h dark, white fluorescent light) for 1 month. In the South (North) site, we used 47 (38) and 56 (35) plants from the Hyogo and Hakodate populations, respectively. We sampled young leaves from one clonal replicate for each parent lines every 2 weeks from 1 September 2011 to 30 August 2012 between 1400 to 1430 hours at the South site. Note that the first sampling on 1 September 2011, at the South site was performed under laboratory conditions. Because all plants from the Hyogo population died in late August 2012 at the South site, we could not collect Hyogo samples for 30 August 2012. At the North site, sampling started after snowmelt on 15 April 2012, and continued until 30 August 2012. The samples were taken from the same plants every 2–10 weeks, depending on the number of surviving replicates per parent line. The leaf samples were immediately preserved either in liquid nitrogen (South site) or in RNAlater solution (North site; Ambion, Foster City, CA, USA). The total number of samples used for gene expression analysis per study site was 254 and 118 with 6 and 2 missing values for the South and North sites, respectively. We recorded the dates of onset of bolting, flowering and reversion. The definitions of the onset of bolting and reversion were the same as for the laboratory experiment. The same plants sampled for gene expression were used for phenology monitoring. Throughout the experiment, the soil surface temperature was recorded every 20 min at the South site using a HOBO Water Temp Pro v2 temperature logger (Onset Computer Corporation, Bourne, MA, USA). At the North site, the soil surface temperature was also recorded every hour using a HOBO H8 Pro temperature logger (Onset Computer Corporation). At both sites, the logger was set just beneath the surface of the soil in the common gardens. Gene expression analysis Total RNA was extracted from 5–10 mg young leaves using an RNeasy Plant Mini Kit (Qiagen, Hilden, Germany) according to the manufacturer’s instructions, followed by DNase treatment using a DNA-free kit (Life Technologies, Grand Island, NY). Complementary DNA was synthesized from 300 ng of total RNA for each sample using a High Capacity RNA-to-cDNA Kit (Life Technologies). The gene expression was measured using real-time PCR with a 7500 fast real-time PCR system and Fast SYBR Green Master Mix (Applied Biosystems). Our real-time PCR experiment included three replicates per sample, and the average was used for analysis. The average expression levels of the target genes were normalized against AhgACTIN2 using the comparative threshold cycle (ΔΔ C t ) method [23] (sequence analysis and primer design are described in the Supplementary Methods ). Modelling gene expression dynamics We propose a kinetic model for AhgFLC and AhgFT expression dynamics on a day-to-day basis with reference to known gene-regulatory dynamics in Arabidopsis. A central gene in the vernalization pathway is FLOWERING LOCUS C ( FLC ), a MADS-domain-containing transcription factor that acts as a floral repressor [11] , [12] by downregulating FLOWERING LOCUS T ( FT ) [16] , [17] . In the photoperiod pathway, the hub gene is CONSTANS ( CO ), which acts as a floral activator by upregulating FT [24] . We formalized the daily dynamics of the AhgFLC and AhgFT expression levels as follows: In equation (1), α FLC ( T ) and β FLC ( T ) describe the production and degradation rates of AhgFLC at the tissue level that are functions of temperature ( T ). Because there was a clear irreversibility in the increase in AhgFLC expression ( Supplementary Fig. S4 ), we added f ( x FLC ), representing the suppression of AhgFLC transcript production at an initial stage after vernalization: where m FLC is the constant that determines the irreversibility of the AhgFLC transcript production. This nonlinearity would be caused by the bistability of FLC on-off dynamics at the cellular level, which is induced by cooperative behaviour in histone modification at the FLC locus (called ‘epigenetic memory’) [25] , [26] . Here, we incorporated the effect of epigenetic memory in a phenomenological manner, but the detailed model of histone modification allows the linking of the mechanism of epigenetic regulation and FLC expression [26] . α FT ( T ) and β FT ( T ) in equation (2), which indicate the production and degradation rates of AhgFT transcript at the tissue level, were both temperature-dependent. The regulation of AhgFT by AhgFLC was formalized using the Hill function g ( x FLC ): where m FT ( T ) is the dissociation constant of AhgFT suppression by AhgFLC (which is temperature-dependent) and H is the Hill constant. The photoperiod effect on AhgFT transcript production was incorporated by h ( ω ): where ω (min) is the photoperiod and is the critical photoperiod above which the AhgFT transcript is produced (the parameter estimation is described in the Supplementary Methods ). Accession codes: The sequence data of AhgVIN3 , AhgFLC and AhgFT have been deposited in UniProt under the accession numbers KC505442-KC505474. How to cite this article: Satake, A. et al . Forecasting flowering phenology under climate warming by modelling the regulatory dynamics of flowering-time genes. Nat. Commun. 4:2303 doi: 10.1038/ncomms3303 (2013).